Impacts of El Niño Southern Oscillation on the global yields of major crops The monitoring and prediction of climate-induced variations in crop yields, production and export prices in major food-producing regions have become important to enable national governments in import-dependent countries to ensure supplies of affordable food for consumers. Although the El Niño/Southern Oscillation (ENSO) often affects seasonal temperature and precipitation, and thus crop yields in many regions, the overall impacts of ENSO on global yields are uncertain. Here we present a global map of the impacts of ENSO on the yields of major crops and quantify its impacts on their global-mean yield anomalies. Results show that El Niño likely improves the global-mean soybean yield by 2.1—5.4% but appears to change the yields of maize, rice and wheat by −4.3 to +0.8%. The global-mean yields of all four crops during La Niña years tend to be below normal (−4.5 to 0.0%). Our findings highlight the importance of ENSO to global crop production. The monitoring and prediction of climate-induced variations in crop yields, production and export prices in major food-producing regions have become increasingly important to enable national governments in import-dependent countries to ensure supplies of affordable food for consumers, including the poor [1] , [2] . Given the high reliability of seasonal El Niño/Southern Oscillation (ENSO) forecasts [3] , [4] , linking variations in global yields with ENSO phase has a potential benefit to food monitoring [5] and famine early warning systems [6] . Although the geographical pattern of the impacts of ENSO on seasonal temperature and rainfall [7] , [8] , and the impacts of ENSO on regional yields [9] , [10] , [11] , are well established, no global map has been constructed to date that describes ENSO’s impacts on crop yields. Only limited information concerning ENSO’s impacts on yields in a few locations is available (for example, in Australia [12] , China [13] , the United States of America [14] , Zimbabwe [15] , Kenya [16] , Indonesia [17] India [18] and Argentina [19] ). Such limited information makes the overall impacts of ENSO on yields that on a global scale are uncertain [20] , and hinders the quantification of the impacts. Although the extent of harvested area also affects crop production, yield is more important in determining production because of the large year-to-year variability of yield associated with climatic factors. Here, we globally mapped the impacts of ENSO on the yields of maize, rice, wheat and soybean. These crops are the principal cereal and legume crops worldwide, providing nearly 60% of all calories produced on croplands [21] . We then quantified ENSO’s impacts on the global-mean yield anomalies of these crops. Our results reveal that ENSO’s impacts on the yields vary among geographical locations, crop types, ENSO phases (El Niño or La Niña) and technology used by the crop-producing regions. The results show that significant negative and positive impacts on the yields associated with El Niño, respectively, appear in up to 22%–24% and 30%–36% of harvested areas worldwide. La Niña has negative impacts on up to 9–13% of harvested areas, with positive impacts being limited to up to 2–4% of harvested areas. El Niño likely improves the global-mean soybean yield but appears to reduce the yields of maize, rice and wheat in most cases, although the magnitude of the impacts varies to some extent by the methods used to calculate normal yield. The global-mean yields of all four crops during La Niña years tend to be below normal. ENSO phases and crop growth cycle In this study, we linked ENSO phases with crop growth cycles. This methodology is illustrated in Fig. 1 that shows whether a key interval that determines crop yield (that is, the reproductive growth period) falls within the phase of El Niño, La Niña or neutral, although the timing of that interval varies by region and crop type ( Supplementary Fig. 1 ). For instance, in 1983, the key growth interval of wheat in the Northern Hemisphere, and in the mid-latitudes in particular, was coincident with El Niño, whereas in the Southern Hemisphere this key growth interval was coincident with La Niña ( Fig. 1a ). We note that the 3-month interval is sufficient to account for the short time-lag of atmospheric teleconnections relative to ENSO sea surface temperature (SST) anomaly. In Goondiwindi, Australia, where a previous study [12] reported large impacts of ENSO on rainfall and wheat crops, below-normal wheat yields often occur during El Niño years, whereas above-normal yields occur in both La Niña years and neutral years ( Supplementary Fig. 2b ). However, the amplitude of the deviation of average positive yield anomalies from normal yields in La Niña years is smaller than that in neutral years ( Supplementary Fig. 2c ). This illustrates the negative impacts of both El Niño and La Niña on wheat yields relative to those yields in neutral years. The amplitude (and even sign) of the average impacts of El Niño and La Niña might vary depending on the methods used to calculate normal yield. We therefore adopted the following two methods: a 5-year running mean ( Supplementary Fig. 2 ) and local polynomial regression ( Supplementary Fig. 3 ), to account for the methodological uncertainty. The small differences between Supplementary Figs 2 and 3 show that the methodological uncertainty is relatively small in terms of the sign of the impacts of ENSO on yield anomalies. 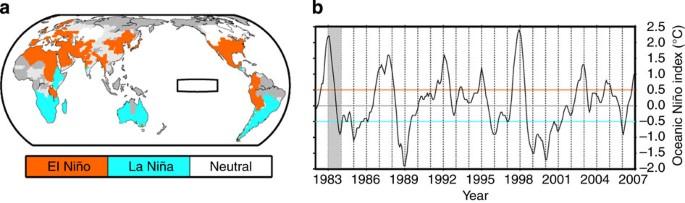Figure 1: Linking the ENSO phase with the key growth interval of a crop. (a) ENSO phase during the reproductive growth period of spring and winter wheat, both harvested in 1983. Light grey indicates that the crop calendar is unavailable, and dark grey designates non-cropland. Only the winter cropping system is presented if both systems are used in a region. The box in the Pacific indicates the Niño3.4 region. (b) Oceanic Niño Index monthly time series; the orange (blue) line indicates the threshold SST of +0.5 °C (−0.5 °C) that categorizes the ENSO phase as El Niño (La Niña), and the grey shaded area indicates the year 1983. Figure 1: Linking the ENSO phase with the key growth interval of a crop. ( a ) ENSO phase during the reproductive growth period of spring and winter wheat, both harvested in 1983. Light grey indicates that the crop calendar is unavailable, and dark grey designates non-cropland. Only the winter cropping system is presented if both systems are used in a region. The box in the Pacific indicates the Niño3.4 region. ( b ) Oceanic Niño Index monthly time series; the orange (blue) line indicates the threshold SST of +0.5 °C (−0.5 °C) that categorizes the ENSO phase as El Niño (La Niña), and the grey shaded area indicates the year 1983. Full size image Geographical distributions of the impacts of El Niño Analyses of yield anomalies (deviations from the 5-year running mean or local polynomial regression curve) from the period 1984–2004 indicate that significant negative impacts of El Niño on the yields are evident in up to 22–24% of harvested areas worldwide ( Fig. 2 and Supplementary Fig. 4 ). The negatively impacted crops and their corresponding regions include the following: maize in the southeastern United States of America, China, East and West Africa, Mexico and Indonesia; soybean in India and in parts of China; rice in the southern part of China, Myanmar and Tanzania; and wheat in a portion of China, the United States of America, Australia, Mexico and parts of Europe. Warmer and drier climate conditions during El Niño years compared with those in neutral years are a primary explanation for the negative impacts of El Niño on the crops in several of the regions listed above, such as maize in Zimbabwe, soybean in India, rice in Indonesia and wheat in Australia ( Supplementary Fig. 5 ), as reported in previous work [9] , [12] , [15] , [17] , [18] . In contrast, significant positive impacts of El Niño on crop yields are found in up to 30–36% of harvested areas worldwide ( Fig. 2 and Supplementary Fig. 4 ), including maize in Brazil and Argentina; soybean in the United States of America and Brazil; rice in part of China, Indonesia and part of Brazil; and wheat in Argentina, Kazakhstan and part of South Africa. Cooler and wetter conditions in these areas during El Niño years ( Supplementary Fig. 5 ) are often correlated with positive impacts on crop yields but with variations across regions and crop types. Negative impacts of El Niño on the yields in irrigated area tend to be mitigated to some extent compared with those in rainfed area ( Supplementary Fig. 6 ). This is because negative impacts of El Niño on the yields in the regions listed above are caused by drier condition. However, the yield data and irrigation map are not always reliable over the interval used in this analysis, and the results for some countries in developing world should be interpreted with caution. 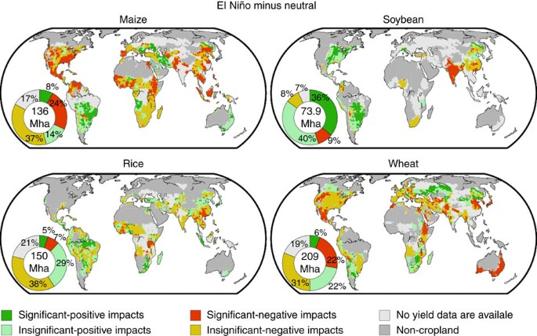Figure 2: Impacts of El Niño on crop yield anomalies for four crops. The 5-year running mean method was used to calculate normal yield. The significance level of the difference in averaged yield anomaly between El Niño years and neutral years was set to be 10% (using the bootstrap with iteration of 10,000 times; the sample size is 7 for El Niño and 8 for neutral years). The pie diagrams indicate the percentages of harvested area in the aforementioned areas. All data in the pie diagrams are normalized to the global harvested area in 2000. Figure 2: Impacts of El Niño on crop yield anomalies for four crops. The 5-year running mean method was used to calculate normal yield. The significance level of the difference in averaged yield anomaly between El Niño years and neutral years was set to be 10% (using the bootstrap with iteration of 10,000 times; the sample size is 7 for El Niño and 8 for neutral years). The pie diagrams indicate the percentages of harvested area in the aforementioned areas. All data in the pie diagrams are normalized to the global harvested area in 2000. Full size image Geographical distributions of the impacts of La Niña The geographical pattern of the impacts of La Niña on the yields is different from that of El Niño. For the four crops examined in this study, significant negative impacts of La Niña appear in part of North, Central and South America, and Ethiopia; and La Niña’s significant positive impacts are found in parts of South and West Africa ( Fig. 3 and Supplementary Fig. 7 ). The negative impacts of La Niña on the yields of maize and soybean in the United States of America are associated with warmer and drier conditions, as previously reported [11] , [14] ( Supplementary Fig. 8 ). Owing to this, the negative impacts of La Niña on these crops and maize particularly in irrigated area tend to be smaller than those in rainfed area ( Supplementary Fig. 6 ). The negatively impacted areas account for up to 9–13% of harvested area worldwide ( Fig. 3 and Supplementary Fig. 7 ). In contrast, the extent of area where significant positive impacts of La Niña are observed is rather limited (up to 2–4% of harvested area worldwide). The percentages of both positively and negatively impacted areas in La Niña years are consistently smaller than the corresponding values in El Niño years ( Figs 2 and 3 , and Supplementary Figs 4 and 7 ). The global crop yields are much more affected both positively and negatively by El Niño than by La Niña. This difference suggests that, in terms of global-mean impacts, the negative impacts of El Niño can be mitigated to some extent by its positive impacts elsewhere, whereas both positive and negative signals of La Niña and their compensation are weaker than those of El Niño. 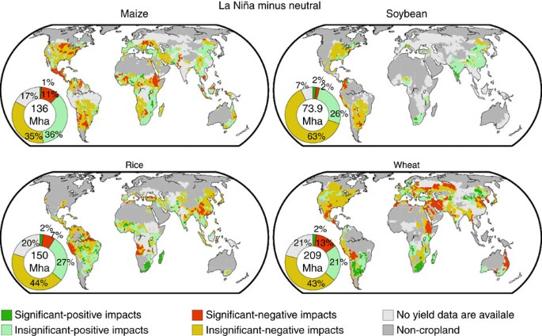Figure 3: Impacts of La Niña on crop yield anomalies for four crops. The 5-year running mean method was used to calculate normal yield. The significance level of the difference in averaged yield anomaly between La Niña years and neutral years was set to be 10% (using the bootstrap with iteration of 10,000 times; the sample size is 6 for La Niña and 8 for neutral years). The pie diagrams indicate the percentages of harvested area in the aforementioned areas. All data in the pie diagrams are normalized to the global harvested area in 2000. Figure 3: Impacts of La Niña on crop yield anomalies for four crops. The 5-year running mean method was used to calculate normal yield. The significance level of the difference in averaged yield anomaly between La Niña years and neutral years was set to be 10% (using the bootstrap with iteration of 10,000 times; the sample size is 6 for La Niña and 8 for neutral years). The pie diagrams indicate the percentages of harvested area in the aforementioned areas. All data in the pie diagrams are normalized to the global harvested area in 2000. Full size image The impacts of ENSO on global-mean yield anomalies The impacts of ENSO on global-mean yield anomalies (weighted by harvested area) vary across crop types, across ENSO phases and across the calculation methods of normal yield. The global-mean yields of maize, rice and wheat in both El Niño and La Niña years tend to be below normal (−4.0 to −0.2%; Fig. 4 and Supplementary Fig. 9 ). Therefore, a decrease in the global production of maize, rice and wheat might be associated with ENSO unless harvested areas and/or the number of harvests in a year increase sufficiently. The global-mean soybean yield in La Niña years tends to be −1.6 to −1.0% below normal. However, the global-mean soybean yield in El Niño years is +2.9 to +3.5% above normal ( Fig. 4 and Supplementary Fig. 9 ). This difference in global-mean yields is caused by the positive impacts of El Niño on crop yields in major crop-producing countries, including the first and second highest soybean-producing countries (the United States of America and Brazil, respectively; Fig. 2 and Supplementary Figs 4 and 10 ). These results indicate that ENSO’s impacts on crop yields form a complex pattern, and that the impacts vary among different geographical locations, different crop types, different ENSO phases, different seasons and different technology adopted by crop-producing areas. Note that although the magnitude of the impacts of ENSO on the yields varies with the analysis methods to some degree, the sign of the impacts is consistent among most methods ( Supplementary Fig. 11 ). 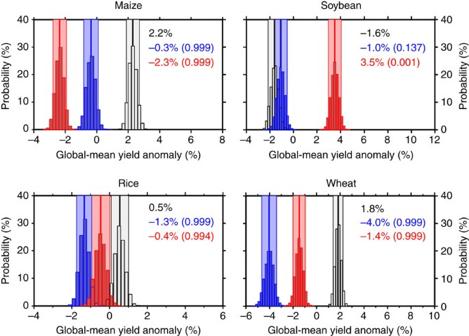Figure 4: Global-mean yield anomalies for four crops during each phase of ENSO. The 5-year running mean method was used to calculate normal yields. Histograms of global-mean yield anomalies (deviations from normal yields) in El Niño years (red), La Niña years (blue) and neutral years (grey). The numbers in each panel are the mean values. The numbers in parentheses indicate the bootstrap probability that the global-mean yield anomaly in El Niño (La Niña) years is lower than that in neutral years. A bootstrap probability value of 0.999 (0.001) indicates a significantly smaller (larger) global-mean yield anomaly in El Niño (La Niña) years compared with that in neutral years at the 0.1% level (using the bootstrap with iteration of 10,000 times). Figure 4: Global-mean yield anomalies for four crops during each phase of ENSO. The 5-year running mean method was used to calculate normal yields. Histograms of global-mean yield anomalies (deviations from normal yields) in El Niño years (red), La Niña years (blue) and neutral years (grey). The numbers in each panel are the mean values. The numbers in parentheses indicate the bootstrap probability that the global-mean yield anomaly in El Niño (La Niña) years is lower than that in neutral years. A bootstrap probability value of 0.999 (0.001) indicates a significantly smaller (larger) global-mean yield anomaly in El Niño (La Niña) years compared with that in neutral years at the 0.1% level (using the bootstrap with iteration of 10,000 times). Full size image Comparisons of this study with previous regional studies Although this study presented the first global map of the impacts of ENSO on yields of the four major crops, there were many similar regional studies [9] , [10] , [11] , [12] , [13] , [14] , [15] , [16] , [17] , [18] , [19] . Supplementary Table 1 shows the comparison of the ENSO’s impacts on the yields revealed in this study and those reported in the previous studies. In general, the signs of the impacts (negative or positive) reported in this study reasonably matches with those reported in the previous studies across the countries and crops despite of some discrepancies ( Supplementary Table 1 ). One example of the discrepancy is the wheat in China. Although the previous study [13] reported that El Niño positively affected the wheat yields in the North China Plain on the basis of the analysis at three sites, our results showed that El Niño has both the positive and negative impacts on the wheat yields in that area ( Fig. 2 and Supplementary Fig. 4 ). The similar discrepancy can be found in the wheat in Argentina ( Supplementary Table 1 ). The previous study [19] reported the positive impacts of El Niño on the wheat yields in the southern part of Argentina and the negative impacts of La Niña on the wheat yields in the northern part of the country based on the county-level yield data. In contrast, our study showed that both the positive and the negative impacts on the wheat yields in Argentine could be seen in both phases of ENSO ( Figs 2 and 3 , and Supplementary Figs 4 and 7 ). The different spatial resolution of yield data between the previous studies and this study (site- or county-level data versus mean yield over a 1.125° grid cell) may help explain these discrepancies. Also the varying length and years of yield data across the studies is another possible reason ( Supplementary Table 1 ). Despite of these discrepancies, however, the overall results of this study are consistent with those of the previous studies. By 2050, the global demand for these major crops is expected to increase by 100–110% from that in 2005 (ref. 21 ). To meet this growing demand, the mean growth rate of global crop production in the coming four decades must reach 2.2–2.4% per year [21] . It is expected that a major portion of this growth will be achieved by an increase in crop yields in areas that have low yields today, which are caused in part by technology that is less able to reduce the impacts of climate variability compared with technology in other areas. Consequently, minimizing the negative impacts of ENSO (for example, the impacts on maize, rice and wheat under El Niño and La Niña) or maximizing the positive impacts of ENSO (for example, the impacts on soybean under El Niño) on global yields are increasingly important not only to ensure short-term food availability but also to maintain positive yield trends. Taking advantage of ENSO’s positive impacts and minimizing its negative impacts might be achieved by basing the choices of planting date, crop type and/or additional inputs of seeds, fertiliser, chemicals and irrigation on the ENSO status or on seasonal climatic forecasts [9] , [10] , [11] , [16] , [22] (for example, http://www.bis.gov.uk/assets/foresight/docs/food-drink/seasonal-weather-forecasting.pdf ). Understanding the contrasting impacts of ENSO on crops in a region, such as the negative impacts on maize yields and the positive impacts on soybean yields in the United States of America under El Niño ( Fig. 2 and Supplementary Fig. 4 ), is useful when making a range of decisions in ENSO-sensitive sectors. Skilful ENSO forecasts have been provided at lead times much longer than those of seasonal temperature and precipitation forecasts [3] . The use of ENSO forecasts is advantageous when linking ENSO forecasts and the impacts of ENSO on crop yields presented here. In addition, the maps presented in this study are useful in the identification of possible regions where weather/crop insurance based on the ENSO index, such as the SST anomaly in Nino3.4 region and its forecasts [1] , [23] (even though seasonal temperature and precipitation forecasts over local regions may be difficult), could be valuable for commercial entities, including farmers. These commercial entities could use this type of insurance to reduce the financial impacts of ENSO-induced decreases in food production. Furthermore, these maps might help reinsurers spread risk across individual insurers in various agricultural regions because several regions are negatively affected by El Niño, whereas different regions are positively affected by El Niño ( Fig. 2 and Supplementary Fig. 4 ). These maps also enable national governments in import-dependent countries to manage regional trade and storage based on the current ENSO phase. Such efforts could increase the ability of national governments and commercial entities in import-dependent countries to effectively respond to ENSO’s impacts on food availability for the poor and could improve farmers’ ability to manage income risk [1] , [23] . An improved response to ENSO could reduce the risk of the population to malnutrition; allow for an increase in agricultural investment in positively impacted years; and improve the adaptation capability to climate variability and change [24] . Finally, increased SST associated with climate change might have gradually modulated ENSO’s behaviour [25] , [26] , [27] , predictability [4] and impacts on the yields. We also note that further assessment is needed for the impacts on yields because of other major climate modes such as the Indian Ocean Dipole [28] , [29] . Existing monitoring and prediction systems for global food security [5] , [6] must be improved to better capture these secular changes. Index of ENSO The Oceanic Niño Index [30] for the period 1982–2006 ( Fig. 1b ), defined as the 3-month running mean of SST anomalies in the Niño3.4 region (5°N–5°S, 120°–170°W; Fig. 1a ), was used to determine whether El Niño or La Niña conditions were present during the reproductive growth period of the four major crops examined in this study. Based on a previous study [2] , the reproductive growth period was specified as a 3-month interval commencing 3 months before harvesting and ending at harvesting. The months of the reproductive growth period were specified in each grid cell using the global crop calendar [31] . Although the climatic conditions during the vegetative growth period are also important, those during the reproductive growth period are factors that more directly determine yields, and thus have been widely used in previous work in the derivation of a climate–crop relationship [2] , [32] . The propagation of the atmospheric Rossby wave (driven by the upper tropospheric divergence forced by the tropical SST anomaly) from the tropics to the mid- to high-latitudes (teleconnection) can finish within a few days. Therefore, in general, monthly mean or seasonal mean is sufficient to account for the time-lag of the atmospheric teleconnections relative to ENSO forcing (note, however, that SST in some remote areas may lag the tropical SST anomaly for a few months because of the large heat capacity of the upper ocean). As noted above, we linked the crop yield anomalies with the Oceanic Niño Index during the 3-month interval, and thus the ENSO teleconnections are well captured in the 3-month mean anomalies. Crop data Grid-cell crop yields for the period 1982–2006 (the grid size is 1.125° in latitude and longitude) were obtained from the satellite statistics-aligned global data set of historical yields [33] , which is a combination of the Food and Agriculture Organization (FAO) of the United Nations country yield statistics and the grid-cell crop-specific net primary production derived from the NOAA/AVHRR (US National Oceanic and Atmospheric Administration/Advanced Very High Resolution Radiometer). These data are therefore estimates of yields rather than observed yields. The reliability of yield estimates was evaluated using the subnational yield statistics in 23 major crop-producing countries [33] and the global data sets of crop yields in 2000 (refs 34 , 35 ). For maize, rice and wheat crops, yields from multiple cropping systems (major/secondary or winter/spring) are available, whereas yields from only a single major cropping system are available for soybean crops. The yield data are not consistently reliable over the analysed time period. The results for some countries in the developing world should be interpreted with caution because the reported production in the FAO statistics on which the grid-cell yields rely may not reflect the actual amount of food available for consumption by people owing to the complexity of accurately monitoring agricultural production and accounting for informal cross-border trade, non-food uses of grain and on-farm wastage [36] . For a given year t , a percentage yield anomaly deviating from a normal yield (defined as a 5-year running mean of yields for the interval t−2 to t+2 or a local polynomial regression curve in a given year t ), , was calculated: where the suffixes t , g and c indicate the year, grid cell and cropping system used for a crop, respectively. Y t, g, c indicates the yield (t ha −1 ), and is the normal yield (t ha −1 ). The calculation of the percentage yield anomalies emphasizes the changes in yields caused by short-term, primarily climate-related factors, although demand, prices, technology and other factors may also affect year-to-year variations in yields. The percentage yield anomalies in the first 2 years (1982 and 1983) and last 2 years (2005 and 2006) were not calculated because the running mean yields for the interval from t−2 to t+2 were not available for those years. The values of the percentage yield anomalies are likely sensitive to the methods used to calculate normal yield. Among other methods for calculating normal yields (for example, Kucharik and Ramankutty [37] ), we used a 5-year running mean method because of the simplicity of this method. We note that the estimated values of global-mean yield anomalies are sensitive to the number of years used for the calculation of normal yield ( Supplementary Fig. 11 ). The general results, however, are similar based on different methods. In addition, we used a local polynomial regression curve fitted to yield time series as the normal yield to account for the uncertainty of yield anomaly values associated with different calculation methods of normal yield. We used ‘Loess’ function in the statistical software R version 2.12.2 (ref. 38 ) with the standard setting of the function (span=0.75, degree=2). When analysing the yield anomalies deviated from the local polynomial regression curve, we did not include the yield anomalies in 1982, 1983, 2005 and 2006 into the analysis; this is to be consistent in the sample size with the analysis using the 5-year running mean method. The calculated percentage yield anomalies were averaged over the period 1984–2004 to obtain an average percentage yield anomaly for each phase of ENSO: where , and are the average percentage yield anomalies (%) in El Niño, La Niña and neutral years, respectively; n El Nino, g , c , n La Nina, g , c and n Neutral, g , c are the number of El Niño, La Niña and neutral years, respectively (that is, n El Nino, g , c + n La Nina, g , c + n Neutral, g , c =21); and ONI t , c is the Oceanic Niño Index value (°C) for the reproductive growth period of the cropping system c of a crop in the year t . The average percentage yield anomalies in El Niño years were further averaged over the cropping systems: where w g, c is the production of the crop of interest using cropping system c (tonnes) and C is the number of cropping systems used to produce each crop of interest. The production yielded by the application of various cropping systems in different countries during the 1990s was obtained from the United States of USA Department of Agriculture (USDA) [39] . The corresponding values for La Niña years ( ) and for neutral years ( ) were calculated in a similar manner. Next the differences between the average percentage yield anomaly in El Niño years and that in neutral years, (%) were computed: The corresponding values for La Niña years ( ) were also computed: Negative (positive) values of and indicate average negative (positive) impacts of El Niño and La Niña on yield anomaly, respectively, relative to average yield anomaly in neutral years. As shown in Supplementary Figs 2c and 3c , the average percentage yield anomalies in both El Niño years and La Niña years in Goondiwindi, Australia, as an example, are smaller than those in neutral years. In this case, the differences between the average percentage yield anomaly in El Niño years and that in neutral years and between the average percentage yield anomaly in La Niña years and that in neutral years are both negative, suggesting negative impacts of El Niño and La Niña on wheat yields in that location, even though the average percentage yield anomaly in La Niña years is above normal. In addition, note that the simple sum of average yield anomaly for the three phases of ENSO ( Supplementary Figs 2c and 3c ) is not necessarily close to zero and their average weighted by the number of years (El Niño, 7; La Niña, 6; and neutral, 8) is theoretically close to zero. The global-mean percentage yield anomaly in El Niño years (relative to the normal yield), (%), was computed using the harvested areas in 2000 (ref. 34 ) as weights: where h g is the grid-cell harvested area of a crop (%) and G is the number of grid cells in which a crop of interest is grown. The global-mean percentage yield anomalies in La Niña years ( ) and in neutral years ( ) were computed in a similar fashion. Positive (negative) values of , or indicate that the global-mean yield is above (below) normal in El Niño, La Nina or neutral years, respectively. Values of are generally expected to be positive because of neutral weather unless yield stagnation or collapse [40] take place. The computed values when using the 5-year running mean method and local polynomial regression method are shown in Supplementary Figs 12 and 13 , respectively. Again, an average of global-mean yield anomalies for El Niño, La Niña and neutral years, weighted by the number of years, is close to zero, but their simple sum is not necessarily close to zero. Climatic data Surface air temperature and soil moisture content of the surface 10-cm layer were obtained from the JRA-25 monthly reanalysis data set [41] . For each cropping system of the four crops analysed in this study, the reanalysis data were averaged over the reproductive growth periods and over the period 1984–2004 to obtain the average temperature during each phase of ENSO: where T El Nino, g, c , T La Nina, g, c and T Neutral, g, c are the average temperatures (°C) during the reproductive growth period in El Niño, La Niña and neutral years, respectively. The temperatures were averaged over the cropping systems of a crop in a similar manner as that described for yields: Similarly, we calculated the average temperatures over the cropping systems of a crop for La Niña years, T La Nina, g , and for neutral years, T Neutral, g . The differences between the average temperature in El Niño years and that in neutral years, ΔT El Nino, g (°C), were then computed: The corresponding temperature values for La Niña years, ΔT La Nino, g , were calculated as follows: Following the procedures described above for temperature, the differences between the average soil moisture content (mm) over the reproductive growth period and over the cropping systems in El Niño years and that in neutral years, ΔS El Nino, g (mm), were calculated. The corresponding soil moisture values for the La Niña years, ΔS La Nino, g , were similarly computed. Thus, the analysis presented here accounted for climatic features specific to individual locations and present over the key growth period. Testing the significance of the impacts of ENSO on yields For each crop, the significance of the difference between the average percentage yield anomaly in El Niño years and that in neutral years, that is, , was tested at each grid cell using the bootstrap method [42] . This calculation procedure is described as follows: (1) For a given crop and grid cell, we pooled the 21 samples of the percentage yield anomaly ( ). Each sample was assigned either an El Niño, La Niña or neutral year according to the Oceanic Niño Index value (ONI t, c ); (2) Values of the percentage yield anomaly in El Niño years were randomly sampled by sampling the number of El Niño years ranging from 1 to n El Nino, g , c : Pooled values of the percentage yield anomaly in El Niño years were averaged over a sampled number of El Niño years to obtain an average percentage yield anomaly in El Niño years ( ). A sample of the average percentage yield anomaly in neutral years ( ) was obtained in a similar manner, using n Neutral, g , c instead of n El Nino, g , c . A sample of the difference between the average percentage yield anomaly in El Niño years and that in neutral years was then computed using an equation combining Equations (5) and (6): (3) The sampling of was iterated 10,000 times, and the number of cases in which the null hypothesis was rejected was counted. The null hypothesis used here was that the difference between the average percentage yield anomaly in El Niño years, and that in neutral years was equal to or greater than zero (that is, ). The ratio between the number of cases in which the null hypothesis was rejected and the total number of sampling iterations corresponded to the bootstrap probability or P value. We set the significance level at 10%. The significance level used here is the same as that used to test the impacts of ENSO on seasonal temperature and precipitation [43] . The significance of the difference between the average percentage yield anomaly in La Niña years, and that in neutral years ( ) was also tested following the above procedures (1) to (3), using n La Nina, g , c instead of n El Nino, g , c . The significance of the differences in the average temperature and in the soil moisture content during the reproductive growth period between El Niño years and neutral years was tested using the same procedures as well. When we tested the significance of the difference between the global-mean percentage yield anomaly in El Niño years and that in neutral years, the calculation procedures (2) and (3) described above were modified as shown below: (2) Sampled values of and were separately averaged across the grid cells and cropping systems using the harvested areas and production shared by cropping system as weights: These calculations correspond to the sampling of the difference between the global-mean yield anomaly in El Niño years and that in neutral years ( ); The sampling of ( ) was iterated 10,000 times, and the number of cases in which the null hypothesis was rejected was counted. The null hypothesis was . We set the significance level at 1%. The significance of the difference between the global-mean yield anomaly in La Niña years and that in neutral years ( ) was tested in a similar manner, using n La Nina, g , c instead of n El Nino, g , c . Different impacts across irrigated and rainfed croplands To survey the potential impacts of irrigation on the impacts of ENSO on crop yields, the global map of monthly irrigated and rainfed crop area in 2000 (ref. 44 ) was used. Using the data, we calculated the percentage of area irrigated (and rainfed) that was located within a 1.125° grid cell for each crop of interest. The mean extent of the irrigated (and rainfed) area was calculated by averaging the monthly data over the entire growth period of a crop of interest, as obtained from the global crop calendar data set [31] . The arranged cells in which the crop was grown were sorted in ascending order, and each top 10% of the irrigated and rainfed areas was categorized as an ‘irrigated area’ or ‘rainfed area,’ respectively. We only used the top 10% samples to avoid cells in which the irrigated and rainfed areas are mixed. These setups are the same with those used in the previous study [2] . We collected the differences in averaged yield anomaly between El Niño (La Niña) years and neutral years over the corresponding cells for each of the two calculation methods of normal yield (the 5-year running mean method and local polynomial regression method). Such data were derived from Figs 2 and 3 ; and Supplementary Figs 4 and 7 . Then, a box plot was provided for each of eight combinations, consisting of two phases of ENSO (El Niño and La Niña), two types of areas (irrigated and rainfed) and two types of methods for calculating normal yield. The provided box plots are presented in Supplementary Fig. 6 . How to cite this article: Iizumi, T. et al. Impacts of El Niño Southern Oscillation on the global yields of major crops. Nat. Commun. 5:3712 doi: 10.1038/ncomms4712 (2014).